Methylome sequencing in triple-negative breast cancer reveals distinct methylation clusters with prognostic value Epigenetic alterations in the cancer methylome are common in breast cancer and provide novel options for tumour stratification. Here, we perform whole-genome methylation capture sequencing on small amounts of DNA isolated from formalin-fixed, paraffin-embedded tissue from triple-negative breast cancer (TNBC) and matched normal samples. We identify differentially methylated regions (DMRs) enriched with promoters associated with transcription factor binding sites and DNA hypersensitive sites. Importantly, we stratify TNBCs into three distinct methylation clusters associated with better or worse prognosis and identify 17 DMRs that show a strong association with overall survival, including DMRs located in the Wilms tumour 1 ( WT1 ) gene, bi-directional-promoter and antisense WT1-AS. Our data reveal that coordinated hypermethylation can occur in oestrogen receptor-negative disease, and that characterizing the epigenetic framework provides a potential signature to stratify TNBCs. Together, our findings demonstrate the feasibility of profiling the cancer methylome with limited archival tissue to identify regulatory regions associated with cancer. Triple-negative breast cancers (TNBCs) comprise a heterogeneous group of cancers with varying prognoses, presenting a challenge for effective clinical management. TNBC is clinically defined by the absence of oestrogen receptor (ER) and progesterone receptor expression, and neither overexpression nor amplification of human epidermal growth factor receptor 2 (HER2) [1] , [2] . TNBC represents ~15–20% of all newly diagnosed breast cancer cases and is generally associated with high risk of disease recurrence and shorter overall survival compared with non-TNBC [3] . Broadly, TNBC patients can be categorized into two distinct groups; those that succumb to their disease within three to five years regardless of treatment and those that remain disease-free to the extent that their overall survival exceeds that of non-TNBC patients (that is, approximately >8 to 10 years post diagnosis) [4] , [5] . Currently, methods by which TNBC patients are stratified into high- and low-risk subgroups remain limited to staging by clinicopathological factors such as tumour size, level of invasiveness and lymph node infiltration. However, unlike other breast cancer subtypes, TNBC outcome is less closely related to stage [6] . Thus, there is a clear need to identify a robust method by which TNBC patients can be stratified by prognosis, to enable more informed disease management. Current efforts to stratify early breast cancer prognosis have primarily focused on multi-gene expression signatures and all have received varying degrees of acceptance [7] . In addition to multi-gene expression assays, DNA methylation signatures are being assessed as potential molecular biomarkers of cancer [8] . A number of studies have documented aberrant methylation events in breast carcinogenesis and identified specific DNA methylation biomarkers that have significant diagnostic and prognostic potential [9] , [10] , [11] , [12] . Several studies have also identified DNA methylation signatures that can distinguish between breast cancer subtypes [13] , [14] , [15] , [16] , and others that may be predictive of treatment response [17] , [18] , [19] . Despite growing interest in the prognostic significance of DNA methylation in breast cancer, there have been no studies specifically investigating the DNA methylation profile of human TNBC and its association with disease outcome. Here we carry out genome-wide DNA methylation profiling of formalin-fixed paraffin-embedded (FFPE) triple-negative clinical DNA samples, using affinity capture of methylated DNA with recombinant methyl-CpG binding domain of MBD2 protein, followed by next generation sequencing (MBDCap-Seq) [20] , [21] . This high-resolution technique allows for genome-wide methylation analysis of CpG rich DNA [22] , [23] . Using MBDCap-Seq, we identify regional methylation profiles specific to TNBC, which we validate using methylation data extracted from TCGA breast cancer cohort [13] . Importantly, we also report the first potential prognostic methylation signature of survival, specific for TNBC that now warrants further study in larger cohorts. Genome coverage of MBDCap-Seq To delineate regions assayable with MBDCap-Seq, we first profiled fully methylated (CpG methyltransferase SssI-treated blood sample) DNA. Computational analysis of SssI MBDCap-Seq revealed that MBDCap-Seq can robustly assess the methylation status of 230,655 regions spanning a total of 116 Mbp, comprising 5,012,633 CpG dinucleotides, or ~18% of the total number of CpG sites in the human genome (see Methods; Supplementary Fig. 1a ). The assayed CpG sites span 91% of all CpG islands; 84% CpG island shores; 72% RefSeq promoters; 38% introns and 31% exons. We next compared coverage of MBDCap-Seq with the Illumina HumanMethylation450K (HM450K) array ( Supplementary Fig. 1b ) and found that MBDCap-Seq interrogates additional 4,740,327 CpG sites as compared with the high-density HM450K array. A major advantage of the MBDCap-Seq method is the ability to interrogate regional blocks of hypermethylation, that is, methylation spanning consecutive CpG sites, which commonly occurs in cancer. We compared regional MBDCap-Seq coverage to coverage of HM450K arrays ( Supplementary Fig. 1a ) and found that while MBDCap-Seq and HM450K arrays have similar regional coverage of CpG islands (91 versus 81%) and RefSeq promoters (71 versus 83%), MBDCap-Seq regional coverage of shores (77 versus 28%), enhancers (12 versus 2%) and insulators (11 versus 1%) is much greater, highlighting the potential advantage of MBDCap-Seq in screening novel functional regions of the cancer methylome. To determine if MBDCap-Seq can also provide accurate methylation analysis from FFPET DNA, we compared DNA methylation profiles from DNA isolated from fresh frozen (FF) and FFPET of matching tumour and lymph node samples. We show that MBDCap-Seq from FFPET provides equivalent methylation to FF DNA (Pearson Correlation Coefficient of 0.95 and 0.86, respectively) ( Supplementary Fig. 2a ) and that MBDCap-Seq and HM450K array performed on the same FFPET tumour and lymph node DNA show high concordance (0.79 and 0.77, respectively) ( Supplementary Fig. 2b–d ). We also show that there are regions uniquely covered by MBDCap-Seq, for example, at enhancers and insulator elements ( Supplementary Fig. 2e,f ). 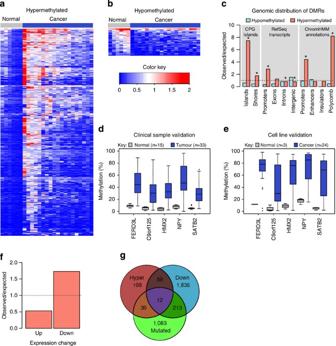Figure 1: MBDCap-seq identifies DMRs in discovery cohort. A heatmap showing methylation profile of 822 hypermethylated (a) and 43 hypomethylated regions (b) across a cohort of 19 tumour and six matched normal samples in the discovery cohort. Columns are samples and rows are regions. The level of methylation (number of reads normalized with respect to fully methylated sample) is represented by a colour scale—blue for low levels and red for high levels of methylation. (c) A bar plot showing association of DMRs across functional/regulatory regions of the genome—(i) CpG islands and shores, (ii) RefSeq transcripts and (iii) Broad ChromHMM HMEC annotation. The height of the bars represents the level of enrichment measured as a ratio between the frequency of hypermethylated (pink) or hypomethylated (blue) regions overlapping a functional element over the expected frequency if such overlaps were to occur at random in the genome. Statistically significant enrichments (Pvalue <0.05; hypergeometric test) are marked with an asterisk. (d) Sequenom validation of five hypermethylated regions—FERD3L,C9orf125,HMX2,NPYandSATB2—is shown for an independent cohort of TNBC samples (normaln=15; tumourn=33) and (e) a panel of breast cancer cell lines (normaln=3; cancern=24). For each region, box plots displaying the distribution of methylation levels are shown in grey/blue for normal/tumour samples/cell lines. (f) A bar plot showing enrichment of genes with promoter hypermethylation in sets of genes that are up-/downregulated in the TCGA cohort of TNBC tumours as compared with matched normal samples. The height of the bars represents the level of enrichment measured as a ratio between the observed number of up-/downregulated genes with promoter hypermethylation to the expected number of such genes. (g) A Venn diagram showing overlap between genes with promoter hypermethylation, genes downregulated in TCGA TNBC cohort (hypergeometric test; FC 1.73;Pvalue≪0.001) and genes with two or more mutations (hypergeometric test; FC 1.92;Pvalue≪0.001) in TCGA breast cancer cohort. Differentially methylated regions in TNBCs To identify differentially methylated regions (DMRs) in TNBCs, we first profiled FFPET DNA using MBDCap-Seq from a discovery cohort of 19 Grade 3 TNBC tumours and six matched normal samples ( Supplementary Table 1 ) and analysed the data with a novel computational pipeline for comparative statistical analysis of MBDCap-Seq samples (see Methods; Supplementary Fig. 3 ). We identified 822 hypermethylated and 43 hypomethylated statistically significant DMRs (FDR <0.05), harbouring 64,005 and 623 CpG sites, respectively, compared with matched normal samples (see Fig. 1a,b ; Supplementary Data 1 ) and validated sample-specific differential methylation using Sequenom DNA methylation analysis ( Supplementary Fig. 4 ). Next, we determined the genomic location of the DMRs and found that CpG islands, CpG island shores and promoters are significantly overrepresented (hypergeometric test; P value <0.0001) in the 822 hypermethylated regions and underrepresented in the 43 regions of hypomethylation ( Fig. 1c ; see Methods). Notably, ChromHMM-annotated HMEC promoters [24] and polycomb repressed regions were also significantly enriched (hypergeometric test; P value ≪ 0.001) for gain of methylation in the breast cancer samples. 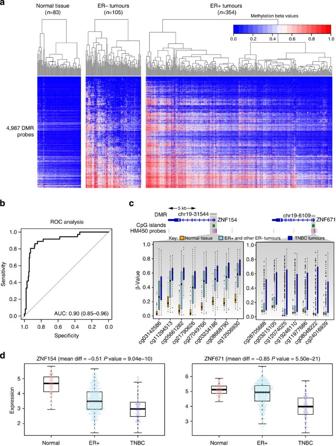Figure 2: Methylation profile of candidate DMRs in the TCGA breast cancer cohort. (a) A heatmap showing methylation profile of TCGA breast cancer samples across 4,987 HM450K probes overlapping hypermethylated DMRs identified in the discovery cohort. Rows are probes and columns are TCGA breast cancer samples profiled on HM450K—83 normal, 105 ER− tumour and 354 ER+ tumour samples. (b) A classifier (Partial Least Squares model) based on methylation values of 282 TNBC-specific probes assigns TCGA HM450K tumour samples into TNBC and non-TNBC with high accuracy; ROC analysis yields AUC of 0.9; assigning samples to highest scoring class (TNBC or non-TNBC) yields sensitivity of 0.72 and specificity of 0.94. The TCGA HM450K cohort was randomly split into training set (TNBCn=37; non-TNBCn=193) and testing set (TNBCn=36; non-TNBCn=193). The model was trained on training set and prediction accuracy assessed on testing set. (c) Box plots showing the distribution of methylation levels for two adjacent regions on chromosome 19 in TCGA normal (n=83), TNBC tumour (n=73), and other breast tumour samples (n=354). These two regions which span the promoters ofZNF154and the adjacentZNF671gene, are hypermethylated in the discovery cohort and exhibit regional TNBC-specific hypermethylation in TCGA cohort, i.e. they are more heavily methylated in TNBC tumours as compared with normal and other tumour subtypes, as shown in the box plots (t-test; mean diff >0.1;Pvalue <0.05). (d) Box plots showing the distribution of expression levels ofZNF154andZNF671genes in TCGA normal (n=92), TNBC tumour (n=119) and ER+ tumour (n=588) samples. The difference in expression of TNBC tumours versus ER+ is significant for both genes (t-test;ZNF154mean diff=−0.51;Pvalue=9.04e−10;ZNF671mean diff=−0.85;Pvalue=5.50e−21). Finally, we validated example DMRs in an independent cohort of 31 TNBCs and 15 normal breast samples and a panel of cell lines ( Supplementary Table 2 ). We performed Sequenom methylation analysis on five of the 822 hypermethylated regions spanning the CpG island promoters of NPY, FERD3L, HMX2, SATB2 and C9orf125 ( Supplementary Fig. 5 ). The levels of methylation detected in the normal samples were uniformly low, whereas the five DMRs showed striking hypermethylation in the TNBCs ( Fig. 1d ) and 24 breast cancer cell lines ( Fig. 1e ). Figure 1: MBDCap-seq identifies DMRs in discovery cohort. A heatmap showing methylation profile of 822 hypermethylated ( a ) and 43 hypomethylated regions ( b ) across a cohort of 19 tumour and six matched normal samples in the discovery cohort. Columns are samples and rows are regions. The level of methylation (number of reads normalized with respect to fully methylated sample) is represented by a colour scale—blue for low levels and red for high levels of methylation. ( c ) A bar plot showing association of DMRs across functional/regulatory regions of the genome—(i) CpG islands and shores, (ii) RefSeq transcripts and (iii) Broad ChromHMM HMEC annotation. The height of the bars represents the level of enrichment measured as a ratio between the frequency of hypermethylated (pink) or hypomethylated (blue) regions overlapping a functional element over the expected frequency if such overlaps were to occur at random in the genome. Statistically significant enrichments ( P value <0.05; hypergeometric test) are marked with an asterisk. ( d ) Sequenom validation of five hypermethylated regions— FERD3L , C9orf125 , HMX2 , NPY and SATB2 —is shown for an independent cohort of TNBC samples (normal n =15; tumour n =33) and ( e ) a panel of breast cancer cell lines (normal n =3; cancer n =24). For each region, box plots displaying the distribution of methylation levels are shown in grey/blue for normal/tumour samples/cell lines. ( f ) A bar plot showing enrichment of genes with promoter hypermethylation in sets of genes that are up-/downregulated in the TCGA cohort of TNBC tumours as compared with matched normal samples. The height of the bars represents the level of enrichment measured as a ratio between the observed number of up-/downregulated genes with promoter hypermethylation to the expected number of such genes. ( g ) A Venn diagram showing overlap between genes with promoter hypermethylation, genes downregulated in TCGA TNBC cohort (hypergeometric test; FC 1.73; P value ≪ 0.001) and genes with two or more mutations (hypergeometric test; FC 1.92; P value ≪ 0.001) in TCGA breast cancer cohort. Full size image Functional characterization of hypermethylated genes To predict the potential functional significance of the 822 DMRs identified in the TNBC, we first determined which regions overlapped with promoters and genes and found that the DMRs were associated with 513 RefSeq promoters, which corresponded to 308 genes ( Supplementary Data 2 ). We used the DAVID functional annotation tool [25] to annotate this set of genes. Visualization of statistically significantly (FDR <0.05) overrepresented gene sets revealed two largely non-overlapping groups of genes [26] (see Methods; Supplementary Fig. 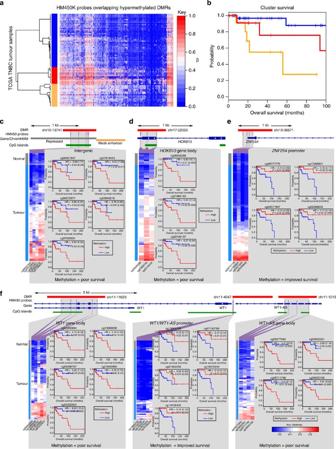Figure 3: Methylation profile stratifies TNBC tumours into survival subgroups. (a) Unsupervised clustering with 4,987 HM450K probes overlapping 822 hypermethylated DMRs identified in the discovery cohort separates TCGA TNBC tumours (n=73) into three main clusters. The heatmap shows the methylation profile of TCGA TNBC tumours and cluster dendrogram. The three clusters are colour-coded with the red cluster exhibiting the highest methylation (TNBC.high), the blue cluster exhibiting the lowest methylation (TNBC.low) and the orange cluster exhibiting an intermediate level of methylation (TNBC.medium). β; methylation beta value. (b) A Kaplan–Meier plot showing survival curves for the patients in the three clusters defined ina. In addition, individual regions of hypermethylation in the discovery cohort overlap with survival-associated probes in the TCGA cohort, including (c) intergenic loci, (d) intragenic loci (for example, theHOXB13gene body) and (e) promoter associate loci (for example,ZNF254promoter). (f) Association with survival for three adjacent regions—chr11-11623, chr11-4047 and chr11-1210—spanning theWT1/WT1-ASlocus is shown. These three regions are hypermethylated in the discovery cohort and overlap several probes showing statistically significant association with overall survival in both univariate and multivariate analyses. For each region, the methylation profile of TCGA TNBC tumour (n=73) and adjacent normal samples (n=9) across overlapping survival probes is shown as a heatmap. The Kaplan–Meier plots for each of the overlapping survival probes is shown as well with corresponding hazard ratios andPvalues from Cox proportional hazards model; values in parentheses correspond to multivariate analysis. HR, hazard ratio. 6 ; Supplementary Table 3 ). One group is annotated with keywords ‘DNA-BINDING’, ‘TRANSCRIPTION’, ‘TRANSCRIPTION REGULATION’, ‘HOMEOBOX’, ‘DEVELOPMENTAL PROTEIN’ and ‘DIFFERENTIATIONS’ and contains approximately 100 genes, mostly transcription factors, such as BARHL2, DLX6, OTX2, RUNX1T1 and TAC1 . The second group is annotated with keywords ‘SIGNAL’, ‘CELL MEMBRANE’, ‘TRANSDUCER’, ‘GLYCOPROTEIN’ and ‘G-PROTEIN COUPLED RECEPTOR’ and contains genes involved in signalling pathways such as ADRB3, GHSR, NPY and ROBO3. To determine whether promoter hypermethylation was potentially involved in gene silencing, we examined TCGA expression data for the 308 genes affected by promoter hypermethylation (see Methods for the analysis of TCGA expression data for TNBC samples; 89 tumour and eight matched normal samples). We found that genes with promoter hypermethylation are enriched in downregulated genes (71 out of 245 genes, for which expression data are available, are downregulated; hypergeometric test; FC 1.73; P value ≪ 0.001) and are depleted in upregulated genes (28 out of 245 genes are upregulated; hypergeometric test; FC 0.53; P value ≪ 0.001) ( Fig. 1f ). To identify potential driver events, we overlapped the 308 hypermethylated genes with genes recurrently mutated in breast cancer in TCGA [13] ( Fig. 1g ). We found that out of 308 genes with promoter methylation, 51 are mutated (hypergeometric test; FC of 1.92; P value ≪ 0.001) and 12 ( C9orf125, COL14A1, ENPP2, ERG2, PLD5, ROBO3, RUNX1T1, SEMA5A, TBX18, TSHZ3, ZBTB16 and ZNF208 ) are both mutated and downregulated. Of these, both ROBO3 and SEMA5A are part of the axon guidance pathway recently implicated in tumour initiation and progression [27] , [28] . Interestingly, promoter hypermethylation affects, in total, seven members of the axon guidance pathway ( CRMP1, GDNF, GFRA1, MYL9, ROBO1, ROBO3 and SEMA5A ) with four members ( GFRA1, MYL9, ROBO3 and SEMA5A ) downregulated. Differentially methylated regions specific to TNBCs We next asked if any of the 822 DMRs were also found in ER− or ER+ breast cancer. We used TCGA breast cancer methylation cohort, which comprises HM450K data for 354 ER+ and 105 ER− breast tumours (73 of which are TNBCs) and 83 normal breast samples (see Methods for the analysis of TCGA methylation data). Of the 822 DMRs regions identified in the MBDCap-seq methylation discovery set, 770 DMRs are interrogated by a total of 4,987 HM450K probes from the TCGA data set. We found that while the majority of these probes are not methylated in breast normal tissue, they were hypermethylated to various degrees in both ER+ and ER− breast cancers ( Fig. 2a ). Both ER+ and ER− subtypes also contained samples with minimal methylation across all probes, as well as those that displayed extensive methylation more representative of a CpG island methylator phenotype (CIMP) [29] . Figure 2: Methylation profile of candidate DMRs in the TCGA breast cancer cohort. ( a ) A heatmap showing methylation profile of TCGA breast cancer samples across 4,987 HM450K probes overlapping hypermethylated DMRs identified in the discovery cohort. Rows are probes and columns are TCGA breast cancer samples profiled on HM450K—83 normal, 105 ER− tumour and 354 ER+ tumour samples. ( b ) A classifier (Partial Least Squares model) based on methylation values of 282 TNBC-specific probes assigns TCGA HM450K tumour samples into TNBC and non-TNBC with high accuracy; ROC analysis yields AUC of 0.9; assigning samples to highest scoring class (TNBC or non-TNBC) yields sensitivity of 0.72 and specificity of 0.94. The TCGA HM450K cohort was randomly split into training set (TNBC n =37; non-TNBC n =193) and testing set (TNBC n =36; non-TNBC n =193). The model was trained on training set and prediction accuracy assessed on testing set. ( c ) Box plots showing the distribution of methylation levels for two adjacent regions on chromosome 19 in TCGA normal ( n =83), TNBC tumour ( n =73), and other breast tumour samples ( n =354). These two regions which span the promoters of ZNF154 and the adjacent ZNF671 gene, are hypermethylated in the discovery cohort and exhibit regional TNBC-specific hypermethylation in TCGA cohort, i.e. they are more heavily methylated in TNBC tumours as compared with normal and other tumour subtypes, as shown in the box plots ( t -test; mean diff >0.1; P value <0.05). ( d ) Box plots showing the distribution of expression levels of ZNF154 and ZNF671 genes in TCGA normal ( n =92), TNBC tumour ( n =119) and ER+ tumour ( n =588) samples. The difference in expression of TNBC tumours versus ER+ is significant for both genes ( t -test; ZNF154 mean diff=−0.51; P value=9.04e−10; ZNF671 mean diff=−0.85; P value=5.50e−21). Full size image Next, we asked whether any of the DMRs were TNBC specific. Out of 4,987 HM450K probes, we found that 5% (282/4,987) were significantly hypermethylated in TNBCs ( t -test; mean differential (diff) methylation >10%; P value <0.05) compared with the ER+ tumours and the rest of the ER−ve tumours. Using methylation values of 282 TNBC-specific probes, we were able to classify tumour samples in the TCGA HM450K cohort into TNBCs and non-TNBCs with sensitivity of 0.72 sensitivity, specificity of 0.94 and AUC 0f 0.90 ( Fig. 2b ). From the 282 TNBC-specific probes, we identified 36 TNBC-specific regions (harbouring at least three or more 450K TNBC-specific probes) that primarily overlap promoters and/or gene bodies ( Supplementary Table 4 ; Supplementary Fig. 7 ). The regions predominantly overlap genes-encoding zinc fingers and transcription factors and intergenic regions that are commonly marked by polycomb in HMECs. An example of two such TNBC-specific regions are located in the promoters of genes-encoding zinc finger proteins ZNF154 and ZNF671 on chromosome 19 ( Fig. 2c ). Both promoters have low methylation levels in normal breast and increased levels of methylation in TNBC samples as compared with ER+ cancer. The distribution of expression values mirrors the methylation status, with normal samples showing the highest levels of expression and TNBC tumours showing the lowest levels of expression ( Fig. 2d ), suggesting silencing by methylation of both ZNF154 and ZNF671 in TNBC tumours. DNA methylation profile can stratify TNBCS To identify DMRs that potentially stratify TNBCs, we used unsupervised cluster analysis on methylation of the 4,987 HM450K probes and identified three distinct groups of TNBC tumours from the TCGA data sets ( Fig. 3a ; see Methods). Survival analysis revealed that the largely hypomethylated cluster (blue cluster) was associated with better prognosis as compared with the other two more highly methylated clusters (orange and red clusters) ( Fig. 3b ). In particular, the medium methylated cluster (orange cluster) comprises samples with the worst prognosis (Cox proportional hazards model; hazard ratio=8.64; P value=0.005) as compared with the good prognosis TNBC cluster (blue cluster). Moreover, there was no association between the induced clusters and survival for ER+ or non TNBC samples ( Supplementary Fig. 8 ). Figure 3: Methylation profile stratifies TNBC tumours into survival subgroups. ( a ) Unsupervised clustering with 4,987 HM450K probes overlapping 822 hypermethylated DMRs identified in the discovery cohort separates TCGA TNBC tumours ( n =73) into three main clusters. The heatmap shows the methylation profile of TCGA TNBC tumours and cluster dendrogram. The three clusters are colour-coded with the red cluster exhibiting the highest methylation (TNBC.high), the blue cluster exhibiting the lowest methylation (TNBC.low) and the orange cluster exhibiting an intermediate level of methylation (TNBC.medium). β; methylation beta value. ( b ) A Kaplan–Meier plot showing survival curves for the patients in the three clusters defined in a . In addition, individual regions of hypermethylation in the discovery cohort overlap with survival-associated probes in the TCGA cohort, including ( c ) intergenic loci, ( d ) intragenic loci (for example, the HOXB13 gene body) and ( e ) promoter associate loci (for example, ZNF254 promoter). ( f ) Association with survival for three adjacent regions—chr11-11623, chr11-4047 and chr11-1210—spanning the WT1/WT1-AS locus is shown. These three regions are hypermethylated in the discovery cohort and overlap several probes showing statistically significant association with overall survival in both univariate and multivariate analyses. For each region, the methylation profile of TCGA TNBC tumour ( n =73) and adjacent normal samples ( n =9) across overlapping survival probes is shown as a heatmap. The Kaplan–Meier plots for each of the overlapping survival probes is shown as well with corresponding hazard ratios and P values from Cox proportional hazards model; values in parentheses correspond to multivariate analysis. HR, hazard ratio. Full size image Next, we determined to what extent regional methylation stratify TNBCs into good and bad prognosis groups. Survival analysis identified 190 probes that were associated with survival in TCGA TNBC samples (Cox proportional hazards model; P value <0.05) in both univariate and multivariate analyses (see Methods). We observed regional association (at least three concordantly located survival probes) for 17 regions; 14 genomic regions with poor survival and three genomic regions for good survival ( Table 1 ; Supplementary Fig. 9 ). Each of the individual Kaplan–Meier plots for individual CpG sites in each region showed excellent survival separation, highlighting the potential value as prognostic biomarkers ( Fig. 3c–e ; Supplementary Fig. 9 ). The genomic location of these regions vary with four regions located in a promoter ( SLC6A3, C6orf174, WT1-AS and ZNF254 ), seven in the gene body only ( DMRTA2, LHX8, WT1, WT1-AS , HOXB13, ECEL1, SOX2-OT ) and five in intergenic regions ( Table 1 ). Interestingly, with the exception of the region encoded by chr10: 102,409,068-102,409,766, all prognostic regions overlap DNase1 hypersensitive sites (ENCODE) and are marked with a polycomb signature in HMEC cells and many contain numerous conserved transcription factor binding sites (TRANSFAC [30] ) ( Table 1 ). Furthermore, we show that the average level of methylation of CpG sites in the 17 potential prognostic regions is higher in the two poor survival groups and is lower in the normal and low-risk groups ( Supplementary Fig. 10 ). Table 1 Summary of 17 DMRs associated with overall survival in TCGA TNBC. Full size table A striking example of regional hypermethylation across consecutive CpG probes that shows statistical significance as a prognostic marker of survival are the DMRs spanning the bi-directional promoter and gene bodies of WT1 gene and its antisense counterpart, WT1-AS ( Fig. 3f ). Wilms tumour protein (WT1) is a zinc finger transcription factor overexpressed in several tumour types including breast [31] . We observe an association between high level of methylation in chr11-11623 and chr11-1210, regions spanning the gene bodies of WT1 and WT1-AS , respectively, and poor survival in TCGA TNBC cohort ( Fig. 3f ). Moreover, increased levels of methylation in these regions are also associated with increased expression of WT1 (chr11-11623) and WT1-AS (chr11-1210) in TNBC patients ( Supplementary Fig. 11 ). Conversely, we observe that TNBC patients with high methylation in chr11-4047, a region spanning bi-directional promoter of WT1 and WT1-AS, survive longer than TNBC patients with low methylation in this region. The prognostic stratification of TNBC patients remains one of the most significant challenges in breast cancer research. While current efforts have primarily focused on the development of multi-gene expression classifiers to inform patient outcome, here we demonstrate the significant prognostic potential of DNA methylation biomarkers for the stratification of TNBCs. We performed genome-wide DNA methylation profiling on TNBC, identified novel regions of differential methylation, and validated regions specific for TNBC using TCGA methylation data as an independent cohort. Strikingly, unsupervised cluster analysis of DMRs stratified TNBC patients into populations of high, medium or low-risk disease outcome. In addition, using both univariate and multivariate Cox proportional hazard models, we identified 17 DMRs significantly associated with TNBC patient survival ( P -value <0.05). Critically, our classifiers paralleled the biologically relevant time-dependent pattern of patient outcome, whereby TNBC patients are most vulnerable to disease-associated death within the first five years following diagnosis, highlighting their potential use as a valuable prognostic application. The DNA methylation aberrations we identified in the TNBC samples follow specific patterns common to many cancer types [32] . For instance, hypermethylation events were localized to CpG islands and shores, while hypomethylation occurred globally across intragenic regions [32] . We observed a strong co-localization of the hypermethylated regions with H3K27me3 marked (polycomb repressed) regions in HMEC cells, supporting the finding that many polycomb-regulated genes are predisposed to aberrant methylation in cancer [33] . We identified 308 genes affected by promoter hypermethylation and functional analysis revealed significant enrichment of genes and transcription factors involved in development and differentiation, as well as DNA binding, homeobox proteins and transcriptional regulation. Hypermethylation of homeobox genes has been previously reported in breast cancer and associated with disease progression and poor patient prognosis [15] , [16] , [34] , [35] . Genes encoding glycoproteins were also enriched in the functional analysis. A significant function of glycoproteins is that of directing immune response [36] . This is particularly poignant since several gene expression modules associated with immune response have been used to predict TNBC patient outcome [37] , [38] , [39] , [40] , [41] . Many of the aberrant cancer promoter hypermethylation events affect genes already silenced in the tissue of origin and therefore considered to be passenger events that do not actively contribute to cancer initiation or progression [42] . To identify potential driver methylation events, we highlighted genes that were both downregulated in TNBC tumours and recurrently mutated in breast cancer. Twelve methylated genes were identified as both mutated and downregulated, including ROBO3 and SEMA5A that are a part of the axon guidance pathway, recently implicated in tumour initiation and progression [27] . In total, promoter hypermethylation affects seven members of the axon guidance pathway. Although the mechanism by which axon guidance drives cancer progression is not completely understood, our data support a potential causal role for DNA methylation for many of these family members in TNBCs. Using an independent TNBC cohort from the TCGA data, we validated 36 TNBC DMRs comprising 20 genes. Strikingly, four of the 20 genes encoded zinc finger proteins (ZNFs). Individual ZNFs and even some clusters of ZNF genes have been found hypermethylated and silenced in several tumour types [43] , [44] , [45] , [46] . In addition, methylation of other ZNF genes have potential prognostic value in prostate and bladder cancer [47] , [48] . Although the mechanisms by which aberrant ZNF expression facilitates oncogenesis are not completely understood, ZNFs are included in two independently derived, TNBC specific, multi-gene expression classifiers (TN45 and Buck 14) [38] , [39] . Recent studies have identified non-TNBC as more heavily methylated compared with TNBC [16] . In our study, we found that a distinct population of both ER+ and ER− tumours are associated with extensive methylation across the DMRs, more representative of a CpG island methylator phenotype (CIMP) [29] . Interestingly, a previous report describes the breast-CIMP (B-CIMP) group comprising solely ER+ tumours [16] ; however, our results show that coordinated hypermethylation can also occur in ER− disease. We also identified three distinct methylation clusters of TNBC tumours based on our DMRs. The largely hypomethylated profile was associated with better survival within the first five years post diagnosis compared with the more heavily methylated subtypes. Interestingly, the medium methylated cluster was associated with the worst survival. Proof of concept that methylation can be used to stratify breast cancer subtypes was recently demonstrated by TCGA, where DNA methylation data were used to classify breast cancer into five distinct subtypes; however, each of the five methylation groups were represented by multiple tumour subtypes and the relationship between methylation and prognosis was not explored [13] . Here, we also identified 17 individual DMRs capable of stratifying TNBC patients into good and poor prognosis groups. Notably, these regions predominately overlap with DNAaseI hypersensitive regions and contain conserved transcription factor binding sites highlighting their potentially significant role in transcriptional regulation. Of the genes listed, many, including WT1, WT1-AS, DMRTA1 and HOXB13, have been previously identified as hypermethylated in numerous cancer subtypes including breast cancer [49] , [50] , [51] , [52] , although associations with patient prognosis were not defined in these studies. Finally, three ‘survival’ DMRs span the bi-directional promoter and gene bodies of WT1 gene and its antisense counter-part WT1-AS . WT1 is an extensively studied transcription factor essential for normal development of the urogenital system and deregulated across many cancer types [31] . In breast cancer, high mRNA levels of WT1 were reported to be associated with poor patient survival [53] and positive modulation of expression of WT1 by its antisense transcript WT1-AS [54] , [55] . Our observed patterns of methylation and survival support an extensive body of evidence on the tight epigenetic transcriptional regulation of WT1 and its role in breast cancer prognosis. More specifically, high levels of methylation across regions spanning gene bodies of WT1 and WT1-AS genes correlate with elevated levels of expression and poor survival, whereas hypermethylation spanning the bi-directional promoter is associated with decreased WT1 and WT1-AS expression and improved survival. Cumulatively, the work presented here highlights the prognostic potential of DNA methylation in TNBC. We identified individual potential biomarkers of patient outcome as well as providing the first evidence to suggest that DNA methylation could be used to stratify TNBC subtypes associated with distinct prognostic profiles. Both observations warrant further clinical investigation in larger independent cohorts as these signatures may in the future provide valuable tools in the management of TNBC. Breast cancer tissue samples Human tissue samples representing normal and tumour breast from fresh frozen and formalin-fixed paraffin-embedded tissue were obtained for this study. Only samples that were classified as triple-negative Grade 3 ductal adenocarcinomas ( Supplementary Table 1 ) were included. The study protocol was approved by the Hunter New England Human Research Ethics Committee (NSW HREC Reference No: HREC/09/HNE/153), Newcastle, New South Wales, Australia and the Princess Alexandra Hospital Human Research Ethics Committee (PAH HREC)(Research Protocol: 2007/165), Brisbane, Queensland. DNA isolation from formalin-fixed paraffin-embedded material DNA isolation from microdissected formalin-fixed paraffin-embedded tissue was performed using the Gentra Puregene Genomic DNA purification tissue kit according to the manufacturer’s instructions (Qiagen). 5 × 1 mm cores or 5 × 10 μm full-faced sections were used for each extraction. The de-paraffinization step was carried out as follows: the paraffin samples were cut into small pieces, 500 μl xylene was added and incubated at 55 °C for 5 min, and the tissue was pelleted at 16,000 g for 3 min, discarding the xylene. After repeating this step, 500 μl 100% EtOH was added for 5 min at room temperature with constant mixing and the tissue collected by centrifugation at 16,000 g for 3 min. The EtOH step was repeated and the tissue pellet dried for 10 min. Then, 300 μl of cell lysis solution was added and the tube incubated for 70 °C for 10 min, followed by the addition of 20 μl Proteinase K (20 mg ml −1 ) to each sample and vortexing for 20 s and incubation in a 55 °C block overnight with constant vortexing. The following day, a further 10 μl proteinase K was added, vortexed for 20 s and further incubated at 55 °C until the samples appear clear. Then, 1 μl RNase A solution (100 mg ml −1 ) was added, mixed by inverting 25 times and incubated at 37 °C for 1 h. The sample was placed on ice to quickly cool it. Then 100 μl protein precipitation solution was added to the cell lysates, vortexed for 20 s, incubated on ice for 5 min and centrifuged at full speed for 5 min at 4 °C to pellet the protein precipitate. The supernatant containing the DNA was carefully removed into a clean microcentrifuge tube. The DNA was precipitated with 300 μl 100% isopropanol, and 2 μl glycogen (20 mg ml −1 ) was added if low yield was expected (<1 μg). The solutions were mixed by inversion (50 times) followed by centrifugation for 10 min at 4 °C. The DNA pellet was washed with 70% EtOH, air-dried and dissolved in 20 μl H 2 O. To dissolve the pellet, it was incubated for 1 h at 65 °C with constant vortexing. Enrichment of methylated DNA by MBDCap The MethylMiner Methylated DNA Enrichment Kit (Invitrogen) was used to isolate methylated DNA from 500 ng to 1 μg of genomic FFPET DNA and was sonicated to 100–500 bp. MBD-Biotin Protein (3.5 μg) was coupled to 10 μl of Dynabeads M-280 Streptavidin according to the manufacturer’s instructions. The MBD-magnetic bead conjugates were washed three times and re-suspended in one volume of 1 × Bind/Wash buffer. The capture reaction was performed by the addition of 500 ng to 1 μg sonicated DNA to the MBD-magnetic beads on a rotating mixer for 1 h at room temperature. All capture reactions were done in duplicate. The beads were washed three times with 1 × Bind/Wash buffer. The bound methylated DNA was eluted as a single fraction with a single high-salt elution buffer (2,000 mM NaCl). Each fraction was concentrated by ethanol precipitation using 1 μl glycogen (20 μg μl −1 ), 1/10 volume of 3 M sodium acetate, pH 5.2 and two sample volumes of 100% ethanol and re-suspended in 60 μl H 2 O. Enrichment of methylated DNA after capture was previously assessed by quantitative PCR of control genes of known methylation status; namely EN1 (heavily methylated) and GAPDH (unmethylated) [22] . Preparation of MBDCap-Seq libraries and Illumina sequencing Ten nanograms of DNA of MBDCap-enriched DNA was prepared for Ilumina sequencing using the Illumina ChIP-Seq DNA sample prep kit (IP-102-1001) according to the manufacturer’s instructions. The library preparation was analysed on Agilent High Sensitivity DNA 1000 Chip. Each sample was sequenced on one lane of the GA11x. Computational analysis of MBDCap-Seq data Sequenced reads were aligned to the hg18 version of the human genome with bowtie. Reads with more than three mismatches and reads mapping to multiple positions were removed. Finally, multiple reads mapping to exactly the same genomic coordinate were eliminated and only one read was retained for downstream analysis. Alignment statistics for samples used in this study are given in Supplementary Table 5 . MBDCap-Seq platform was previously shown to interrogate CpG dense regions of the genome [23] . To accurately delineate regions of the genome assayable by MBDCap-Seq, we used fully methylated sample (SssI blood sample) to guide us to the genomic regions attracting sequenced tags. More specifically, we applied findPeaks peak calling utility from HOMER suite of programs [56] to fully methylated sample (with parameter settings of -style histone -size 300 -minDist 300 -tagThreshold 18) to identify 230,655 regions covering ~116 Mbp of the genome. We interchangeably refer to these regions as regions of interest or SssI regions. For each MBDCap-Seq sample to be analysed, we computed the number of sequenced tags overlapping SssI regions, which resulted in table of counts where columns are samples and rows are SssI regions. We used edgeR Bioconductor package [57] ( http://www.bioconductor.org/packages/release/bioc/html/edgeR.html ) to model distribution of reads between normal ( n =6) and tumour ( n =19) group of samples in the discovery cohort. Since edgeR package does not support modelling of paired and unpaired data simultaneously, we performed two separate analyses, a paired analysis with six normal/tumour pairs and unpaired analysis with all the samples, and then intersected the results. We found 822 hypermethylated and 43 hypomethylated regions at FDR threshold of 0.05 in both paired and unpaired analyses. Clustering of MBDCap-Seq data The number of reads mapping to a particular region of genome depends not just on the average level of methylation in the region, but also on other factors, such as density of methylated CpG nucleotides. To compare MBDCap-Seq readout to other more quantitative technologies such as HM450K and Sequenom, we used fully methylated MBDCap-Seq sample to normalize MBDCap-Seq readouts for samples in the discovery cohort. More specifically, let X i be the number of tags overlapping region i and N be the total number of tags overlapping SssI regions in the sample to be normalized and Y i and M be the corresponding numbers in the control sample. Then, the normalized number of tags overlapping the region i is given by We used normalized tag counts for heatmap visualization in Fig. 1 , for comparison with HM450K in Supplementary Fig. 2 , and for comparison with Sequenom in Supplementary Fig. 4 . Functional annotations of the genome CpG island annotation for hg18 was obtained from UCSC genome browser. The location of CpG island shores was derived from CpG islands by taking ±2 Kb flanking regions and removing any overlaps with CpG islands. RefSeq transcript annotation for hg18 was obtained from UCSC genome browser. Promoters were defined as +2,000/−100 bp around transcription start site. Intergenic regions were defined as regions complementing transcript regions extended to ±2 Kb around the transcripts. HMEC ChromHMM annotations for hg18 were downloaded from ENCODE. The original annotation partitions the HMEC genome into 15 functional states (see Fig. 1b in ref. 24 ). In Fig. 1c and Supplementary Fig. 1B , for brevity, we collapsed the three original promoter states into one promoter state and the four original enhancer states into one enhancer state. Enrichment analysis statistical methods For the enrichment analysis of hypermethylated regions, we used hypergeometric test to assess the enrichment of various functional annotations of the genome in the set of differentially methylated regions. For a given functional annotation represented by a set of genomic regions, fraction of SssI regions (regions assayable by MBDCap-Seq) overlapping functional annotation was compared with the fraction of hyper-/hypomethylated regions overlapping functional annotation using hypergeometric distribution. For the enrichment analysis of genes affected by promoter hypermethylation, first, we used DAVID functional annotation tool [25] to carry out analysis against gene sets defined by SP_PIR_KEYWORDS annotation. Second, we used hypergeometric test to assess the enrichment of additional gene sets in the set of genes affected by promoter hypermethylation [26] . In both the analyses, the set of 15,643 RefSeq genes with promoters overlapping SssI regions was used as a background. Sequenom quantitative massARRAY methylation analysis Sequenom MassARRAY methylation analysis was performed according to Coolen et al. [58] Briefly, 500 ng of FFPET clinical sample and cell line DNA ( Supplementary Table 2 ) was extracted and bisulphite treated using the standard bisulphite protocol [59] . As controls for the methylation analysis, whole-genome amplified DNA (0% methylated) and M.SssI-treated DNA (100% methylated) were bisulphite treated in parallel. The primers were designed using the EpiDesignerBETA software from Sequenom (see Supplementary Table 6 for sequences). Each reverse primer has a T7-promoter tag (5′-CAGTAATACGACTCACTATAGGGAGAAGGCT-3′) and each forward primer has a 10-mer tag (5′-AGGAAGAGAG-3′). On testing these primers on bisulphite-treated DNA, all the primers gave specific PCR products at a Tm of 60 °C. To check for potential PCR bias towards methylated or non-methylated sequences, we used serological DNA (Millipore) as a 100% methylated control and whole-genome amplified human blood DNA as a 0% methylated control. The PCRs were optimized and performed in triplicate using the conditions: 95 °C for 2 min, 45 cycles of 95 °C for 40 s, 60 °C for 1 min and 72 °C for 1 min 30 s and final extension at 72 °C for 5 min. After PCR amplification, the triplicates were pooled and a shrimp alkaline phosphatase treatment was performed using 5 μl of the PCR product as template. Then, 2 μl of the shrimp alkaline phosphatase-treated PCR product was taken and subjected to in vitro transcription and RNaseA Cleavage for the T-cleavage reaction. The samples were purified by resin treatment and spotted on a 384-well SpectroCHIP by a MassARRAY Nanodispenser. This was followed by spectral acquisition on a MassARRAY Analyser Compact matrix-assisted laser desorption/ionization time-of-flight mass spectrometry. The results were then analysed by the EpiTYPER software V 1.0, which gives quantitative methylation levels for individual CpG sites. The average methylation ratio was calculated by averaging the ratios obtained from each CpG site. For the Sequenom validation, sample sizes were determined for a two sample t -test with a two-sided alpha of 0.01, assuming five regions were to be investigated. Assuming the difference in average methylation levels is 0.25 (tumour: s.d.=0.2, normal: s.d.=0.05), to have 90% power to establish a significant difference between tumour and normal samples, 15 samples per group were required. The calculations are based on preliminary data from the lab on methylation levels in breast cancer and normal samples (unpublished). Acquisition of TCGA data Throughout the paper, we used several molecular data sets from TCGA breast cancer (BRCA) cohort. Clinical annotation of samples was obtained from the marker TCGA BRCA publication (Supplementary Table 1 in ref. 13 ; Supplementary Table 7 ). Raw HM450K methylation data (Level 1) was obtained from TCGA data portal in January 2012. Methylation data spanned 67 normal and 354 tumour ER+ samples, 16 normal and 105 tumour ER− samples and nine normal and 73 tumour TNBC samples. Processed array expression data (Level 3) was obtained from TCGA data portal in March 2012. Expression data spanned 52 normal and 406 tumour ER+ samples, nine normal and 118 tumour ER− samples and eight normal and 89 tumour TNBC samples. Processed RNA-Seq expression data (Level 3) were obtained from TCGA data portal in December 2012. Expression data spanned 73 normal and 588 tumour ER+ samples, 19 normal and 174 tumour ER− samples and 12 normal and 119 tumour TNBC samples. Summary of TCGA BRCA mutation data was obtained from COSMIC database ( http://cancer.sanger.ac.uk/cosmic/study/overview?study_id=414 ). The summary lists mutations in gene coding regions across patients including both synonymous and non-synonymous amino-acid substitutions. We consider a gene as mutated if it appears at least two times in the list ( Supplementary Table 8 ). Analysis of HM450K methylation data The raw HM450K data were preprocessed and background normalized with Bioconductor minfi package using preprocessIllumina(..., bg.correct=TRUE, normalize=`controls', reference=1) command; resulting M-values were used for statistical analyses [60] and beta-values for heatmap visualizations and clustering. To identify TNBC-specific HM450K probes, we carried out t -test comparison between TNBC ( n =73) and non-TNBC ( n =386) tumours. This analysis resulted in 282 probes having adj. P value <0.05 and estimated mean difference of methylation between TNBC and non-TNBC tumours of at least 10%; these probes were declared as TNBC specific. Regions overlapping three or more TNBC-specific probes were declared as TNBC specific. For TNBC-specific signature, we trained a Partial Least Squares model as implemented in the caret R package [61] , [62] to classify tumours into TNBC and non-TNBC based on the methylation values of 282 TNBC-specific probes. The tumour samples in the TCGA HM450K cohort were randomly partitioned into equal-size training/testing sets. The model parameters were derived from training set and then applied to make predictions on the testing set. The performance of the model was assessed using test set predictions. Analysis of expression data Differential expression analysis between normal ( n =8) and tumour ( n =89) TNBC samples was carried out with Bioconductor limma package. Since only subset of tumour samples had paired adjacent normal samples, patient data were treated as random effect using limma’s duplicateCorrelation(…) function. This analysis resulted in 3,017 downregulated and 3,407 upregulated genes with adj. P value <0.05 out of 17,655 genes on the array. In Fig. 1f,g , we only considered genes with SssI regions in their promoter regions reducing the number of downregulated, upregulated and total genes to 2,119, 2,722 and 15,543, respectively. We used log-transformed RNA-Seq expression values to highlight the relationship between methylation and expression for number of candidate regions in Fig. 2c and Supplementary Fig. 11 . Survival analysis TNBC tumour samples in TCGA HM450K cohort ( n =73) were clustered on the basis of methylation beta-values of 4,987 HM450K probes overlapping the 822 hypermethylated regions. We applied consensus clustering algorithm [63] as implemented in Bioconductor ConsensusClusterPlus package to the 4,987 × 73 methylation matrix with parameters maxK=4, reps=1000, pItem=0.8, pFeature=0.8, clusterAlg=`km', distance=`euclidean'. We used SVD decomposition to reduce the dimension of the methylation matrix to R 10 before clustering. We chose the three-cluster configuration for downstream survival analysis. Survival analysis was carried out using Cox proportional hazards model as implemented in R survival package against overall survival data ( Supplementary Table 7 ). Survival analysis of cluster data was carried out with cluster membership as an explanatory variable. The BRCA TNBC cohort consists of 73 patients with HM450K methylation data and 12 events. Survival analysis of individual probes (4,987 probes overlapping 822 hypermethylated DMRs) was carried out with probe methylation status as explanatory variable (univariate analysis) and age, stage and probe methylation status (multivariate analysis). Methylation status was represented by a binary variable, high (higher than the median beta-value for the probe) and low (smaller or equal to the median beta-value for the probe). Stage was derived from AJCC stage in the clinical annotation of samples. Due to moderate size of the cohort, we reduced the number of values of the stage variable to two by collapsing stages I, IA, IB, II, IIA and IIB into one state and stages III, IIIA, IIIB, IIIC and IV into one state. This resulted in 190 probes with methylation status statistically and significantly ( P value <0.05 in both univariate and multivariate analyses) associated with overall survival in TCGA TNBC patients. Regional aggregation of survival probes identified 17 hypermethylated DMRs overlapping three or more survival probes. Fourteen regions were associated with poor prognosis, these regions overlapped probes for which high methylation corresponded to lower probability of survival, and three regions were associated with good prognosis. How to cite this article: Stirzaker, C. et al. Methylome sequencing in triple-negative breast cancer reveals distinct methylation clusters with prognostic value. Nat. Commun. 6:5899 doi: 10.1038/ncomms6899 (2015). Accession codes: Methylation sequence data have been deposited in GenBank/EMBL/DDBJ under the accession code GSE58020.